Microorganisms from aphid honeydew attract and enhance the efficacy of natural enemies Aphids are one of the most serious pests of crops worldwide, causing major yield and economic losses. To control aphids, natural enemies could be an option but their efficacy is sometimes limited by their dispersal in natural environment. Here we report the first isolation of a bacterium from the pea aphid Acyrthosiphon pisum honeydew, Staphylococcus sciuri , which acts as a kairomone enhancing the efficiency of aphid natural enemies. Our findings represent the first case of a host-associated bacterium driving prey location and ovipositional preference for the natural enemy. We show that this bacterium has a key role in tritrophic interactions because it is the direct source of volatiles used to locate prey. Some specific semiochemicals produced by S. sciuri were also identified as significant attractants and ovipositional stimulants. The use of this host-associated bacterium could certainly provide a novel approach to control aphids in field and greenhouse systems. Aphids are pests that, by their rapid growth and their ability to spread, constitute major problems for crop production [1] . The use of chemical treatments, unfortunately still widespread, leads to the selection of resistant individuals whose eradication becomes increasingly difficult [2] , [3] , [4] , [5] . Natural enemies such as predators and parasitoids could be an option [6] , [7] , [8] , [9] , but their efficacy is sometimes limited by their dispersal in natural environment as they are generally highly mobile insects. When feeding on the plant phloem sap, aphid excretes large amounts of honeydew, a complex mixture of sugars, organic acids, amino acids and some lipids [10] , [11] , [12] . The composition of honeydew is driven by the host plant that the aphid is feeding on but also by the aphid itself, including its primary symbionts. Indeed, sugars and amino acids found in the honeydew reflect the phloem sap composition [12] but additional sugars are also synthesized by the sap feeder [10] . Essential amino acids are also provided by endosymbiotic bacteria to correct the very low and unbalanced concentrations of amino acids in the phloem sap [13] , [14] . This excretory product is considered as a food complement for many aphid natural enemies [15] , [16] , [17] and the volatiles that are released are supposed to act as kairomones for parasitoids and predators [18] , [19] , [20] , [21] , [22] , [23] , [24] . However, the identification of the semiochemicals or volatiles released from natural honeydew has not yet been established [25] . Because honeydew is mainly composed of sugars and amino acids, this excretion constitutes an excellent growth medium for microorganisms that actively contribute to the production of volatile compounds [26] . Many investigations using gas chromatography and mass spectrometry have illustrated the ability of bacteria to produce volatile compounds [27] , [28] , [29] ; however, their ability to attract insects has been demonstrated in only a very few studies [30] , [31] , [32] , [33] . In biological control, bacterial volatile compounds can serve as signals and act as semiochemicals, attracting or repelling different insects [27] . Among aphids' enemies, the hoverfly Episyrphus balteatus (De Geer) (Diptera: Syrphidae) is recognized as a very efficient aphidophagous predator. This syrphid is considered as the most abundant natural enemy in agroecosystems and natural habitats [34] , [35] , as the most efficient aphid predator [36] and is associated with many different aphid-plant complexes [37] . Furthermore, E. balteatus larvae feed on a large variety of aphid species and are voracious feeders, often eating hundreds of aphids during their development [38] . At the adult stage, they have an excellent efficiency in locating aphid colonies, using both vision and semiochemicals released from their prey or from infested plants [23] , [38] , [39] . Here we show that a bacterium from the microflora of the pea aphid A. pisum honeydew (a host-associated bacterium) produces semiochemicals that act as effective attractants and ovipositional stimulants for the hoverfly E. balteatus . These findings could lead to the generation of new methods for aphid biological control. Identification of the honeydew volatile compounds Because honeydew was suspected to emit semiochemicals, volatiles from honeydew samples were collected by solid-phase microextraction (SPME) and analysed by gas chromatography-mass spectrometry (GC–MS). 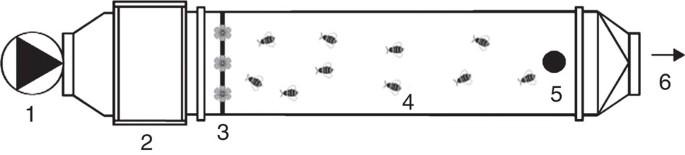Figure 1: Wind tunnel to record theE. balteatusbehaviours in response to honeydews and semiochemicals. Experimental setup of the wind tunnel used to record behaviours. 1, Fan; 2, Filters; 3,V. fabaplants; 4, hoverflies; 5, hoverflies release point; 6, wind direction. Fifteen volatiles were identified from crude honeydew including alcohols, ketones, aldehydes, a pyrazine, a monoterpene and acids ( Table 1 ). Table 1 Honeydew volatile compounds. Full size table Origin of the volatile compounds Because of the possible sources of volatile compounds could be bacterial, a global study of the pea aphid ( A. pisum ) honeydew flora was conducted. Two cultivable bacteria were isolated and identified by 16S ribosomal DNA sequences as Staphylococcus sciuri (Bacilles: Staphylococcaceae) and Acinetobacter calcoaceticus (Pseudomonadales: Moraxellaceae). The prevalences of the two strains were respectively 3×10 6 and 9×10 6 CFU per ml. Because S. sciuri has been previously found from gut flora of some laboratory aphid species and to verify whether this bacterium as well as A. calcoaceticus are present in the honeydew flora of wild aphids, the honeydew flora of ten aphid natural species was analysed ( Supplementary Table S1 ). S. sciuri was isolated from two aphid species: Macrosiphum euphorbiae (Thomas) feeding on Cucurbita pepo L. (1×10 3 CFU per ml) and Amphorophora idaei (Börner) feeding on Rubus idaeus L. (2×10 3 CFU per ml). The bacterium A. calcoaceticus was identified from one aphid species: Aphis fabae (Scopoli) feeding on Carduus nutans (Nyman) (1×10 4 CFU per ml). These results indicated that S. sciuri and A. calcoaceticus occur naturally among natural aphid populations and that these bacteria are not contaminants from laboratory handlings. To determine whether bacteria were responsible for the emission of semiochemicals, SPME and GC–MS analyses were performed on different honeydew samples. Only a few volatiles were detected when the honeydew was filtered to eliminate the bacteria, or when sterile honeydew was reinoculated with the A. calcoaceticus bacterium ( Table 1 ). However, nearly all the volatiles previously found in crude honeydew were detected in the honeydew reinoculated with S. sciuri ( Table 1 ). When the 863 medium was inoculated with the S. sciuri bacterium, the same results were obtained because most of the crude honeydew volatile compounds were detected ( Table 1 ). This strongly indicated that the active honeydew volatiles are mainly produced by S. sciuri . Origin of S. sciuri and A. calcoaceticus identified from the honeydew Because the origin of the bacteria identified from the honeydew could be the aphids themselves or the surrounding environment, the occurrence of S. sciuri and A. calcoaceticus in the body of the pea aphid ( A. pisum ) was checked. After isolation, the two bacteria S. sciuri and A. calcoaceticus were identified by 16S ribosomal DNA sequences. The prevalences of the two strains in the aphid body were, respectively, 2×10 6 and 8×10 6 CFU per ml. Effects of the identified semiochemicals on hoverflies To determine whether the presence of bacteria in aphid honeydew and the identified semiochemicals have a real impact on natural enemy behaviour, wind tunnel assays were performed with the hoverfly E. balteatus ( Fig. 1 ). Wind tunnel assays enable direct observations of the upwind attraction response under controlled stimulus and environmental conditions [40] , [41] . Although the filtered and the A. calcoaceticus -reinoculated honeydews directly sprayed on plants did not affect the syrphid behaviour, crude honeydew and S. sciuri -reinoculated honeydew had a significant impact on the foraging and oviposition behaviour of the hoverflies. Indeed, when non-infested plants were sprayed with crude honeydew, nearly half (48±3%) of the tested hoverflies were observed near (less than 30 cm) the plants (attraction) with 27±2% of them on the plants ( Fig. 2a ; Supplementary Table S2 ). In addition, 46±3% of hoverflies that approached treated plants remained around them (less than 30 cm) throughout the observation time (retention). Similar behaviours were adopted by insects when plants were sprayed with the S. sciuri -reinoculated honeydew (attraction: 47±2% of individuals; retention: 43±3% of individuals; 28±2% of individuals on the plants) ( Fig. 2a ; Supplementary Table S2 ). Both crude (58±3 eggs) and S. sciuri -reinoculated honeydew (63±6 eggs) treatments strongly stimulated oviposition and gave an identical number of eggs than that obtained with the positive control (plants infested with aphids) (65±9 eggs) ( Fig. 2b ; Supplementary Table S2 ). Figure 1: Wind tunnel to record the E. balteatus behaviours in response to honeydews and semiochemicals. Experimental setup of the wind tunnel used to record behaviours. 1, Fan; 2, Filters; 3, V. faba plants; 4, hoverflies; 5, hoverflies release point; 6, wind direction. 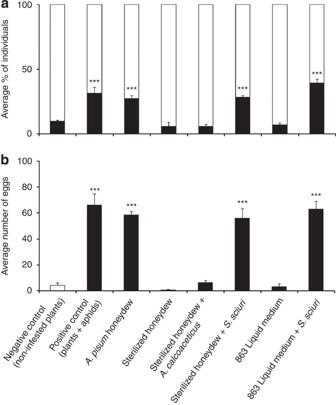Figure 2: Attraction on the plants and oviposition ofE. balteatus. Behavioural responses to the 863 medium, 863 medium inoculated withS. sciuri, crude honeydew, sterilized honeydew or sterilized and then reinoculated honeydew. (a) Average percentage of individuals recovered on the plants (in black on the graph) and elsewhere in the wind tunnel (n=20×6 observations). (b) Average number of eggs on plants after 120 min (n=20). ***indicates significant difference with the control atP<0.001 (generalized Linear Mixed Models). Error bars indicate standard errors. Full size image Figure 2: Attraction on the plants and oviposition of E. balteatus . Behavioural responses to the 863 medium, 863 medium inoculated with S. sciuri , crude honeydew, sterilized honeydew or sterilized and then reinoculated honeydew. ( a ) Average percentage of individuals recovered on the plants (in black on the graph) and elsewhere in the wind tunnel ( n =20×6 observations). ( b ) Average number of eggs on plants after 120 min ( n =20). ***indicates significant difference with the control at P <0.001 (generalized Linear Mixed Models). Error bars indicate standard errors. Full size image Volatiles previously identified from A. pisum honeydew were then tested individually. Three volatiles attracted E. balteatus : 3-methyl-2-butenal, 3-methylbutanoic acid and 2-methylbutanoic acid attracted respectively 23±4, 22±3 and 23±3% of individuals on the plants ( Fig. 3a ; Supplementary Table S2 ). Two of these volatiles also induced E. balteatus oviposition ( Fig. 3b ; Supplementary Table S2 ): 3-methyl-2-butenal led to an identical number of eggs (59±4 eggs) to that found for the positive control (65±9 eggs) and a considerable number of eggs were obtained with 2-methylbutanoic acid (18±4 eggs). If butanoic acid only attracted 8.0±1% of individuals ( Fig. 3a ; Supplementary Table S2 ), this volatile also induced the oviposition because 14±5 eggs were laid on the plants ( Fig. 3b ; Supplementary Table S2 ). Among the 15 volatiles tested, 3-methyl-2-butenal and 2-methylbutanoic acid, acting as attractants and as ovipositional stimulants, were produced by the S. sciuri strain as they were not detected with the filtered honeydew. 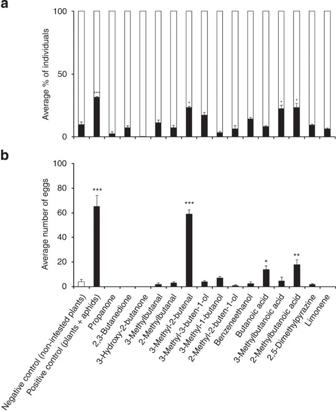Figure 3: Attraction on the plants and oviposition ofE. balteatus. Behavioural responses to semiochemicals from theA. pisumhoneydew. (a) Average percentage of individuals recovered on the plants (in black on the graph) and elsewhere in the wind tunnel (n=20×6 observations). (b) Average number of eggs on plants after 120 min (n=20). *, **and ***, respectively, indicate significant difference with the control atP<0.05,P<0.01 andP<0.001 (generalized linear mixed models). Error bars indicate standard errors. Figure 3: Attraction on the plants and oviposition of E. balteatus . Behavioural responses to semiochemicals from the A. pisum honeydew. ( a ) Average percentage of individuals recovered on the plants (in black on the graph) and elsewhere in the wind tunnel ( n =20×6 observations). ( b ) Average number of eggs on plants after 120 min ( n =20). *, **and ***, respectively, indicate significant difference with the control at P <0.05, P <0.01 and P <0.001 (generalized linear mixed models). Error bars indicate standard errors. Full size image The concentrations of 3-methyl-2-butenal, butanoic acid and 2-methylbutanoic acid were, respectively, 0.394±0.014, 0.126±0.011 and 0.023±0.008 ng μl −1 in crude honeydew and 0.354±0.098, 0.189±0.015 and 0.024±0.009 ng μl −1 in the S. sciuri -reinoculated honeydew ( Table 2 ). Table 2 Quantification of honeydew volatile compounds. Full size table Effects of the S. sciuri culture medium on hoverflies To determine whether the bacterium S. sciuri could be used directly in biological control, the culture medium (863 medium) of S. sciuri was tested as an attractant. Assays in the wind tunnel showed that the culture medium of S. sciuri induced the same behaviours than those observed with crude honeydew sprayed on plants: 55±1% of individuals were attracted, 39±1% were found on the plants ( Fig. 2a ; Supplementary Table S2 ), and the oviposition (56±7 eggs) was equal to that obtained in natural conditions (plants+aphids) ( Fig. 2b ; Supplementary Table S2 ). The non-inoculated 863 medium did not attract the hoverflies, confirming the surprising role that this bacterium had. The concentrations of 3-methyl-2-butenal, butanoic acid and 2-methylbutanoic acid were, respectively, 0.348±0.090, 0.145±0.031 and 0.029±0.004 ng μl −1 in the culture medium (863 medium) of S. sciuri , whereas these volatiles were not detected in the non-inoculated 863 medium ( Table 2 ). To validate the laboratory observations, the culture medium of S. sciuri was first tested under a greenhouse. In the area treated with the 863 medium, an equivalent number of eggs (3±0.7 eggs) was counted on the plants when compared with the untreated area (1±0.1 eggs) ( Fig. 4a ; Supplementary Table S3 ). When the culture medium of S. sciuri was sprayed on plants, a higher number of 8±2 eggs per plant were observed in the treated area in comparison with the untreated area (2±0.3 eggs) ( Fig. 4b ; Supplementary Table S3 ). This indicates that the bacterium S. sciuri rather than the 863 medium significantly induced the oviposition. Secondly, the biological effect of the S. sciuri culture medium was evaluated in a potato field: the parcels sprayed with this formulation clearly attracted a high number of hoverflies (11±3 individuals per m 2 ) in comparison with the untreated areas (3±0.5 individuals per m 2 ) ( Fig. 5a ; Supplementary Table S4 ). The areas treated with the 863 medium did not attract more hoverflies (5±1 individuals per m 2 ) than the untreated areas (3±0.5 individuals per m 2 ) ( Fig. 5a ; Supplementary Table S4 ). Significantly more syrphid eggs were also observed on the plants treated with the culture medium of S. sciuri (28±4 eggs per m 2 ) in comparison with the non-treated plants (6±1 eggs per m 2 ) ( Fig. 5b ; Supplementary Table S4 ), and the 863 medium did not stimulate the oviposition (5.5±1 eggs per m 2 ) in comparison with the untreated plants (6±1 eggs per m 2 ) ( Fig. 5b ; Supplementary Table S4 ). Once again, the field experiments highlighted the key role that S. sciuri had both for attraction and oviposition stimulation. 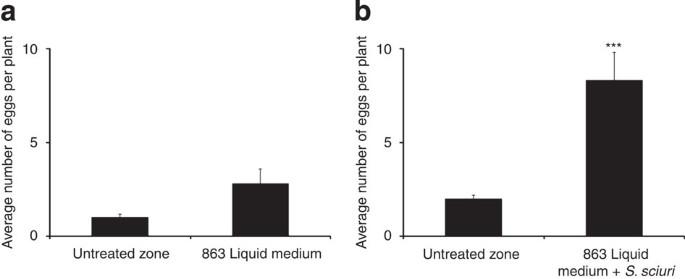Figure 4: Effect of the 863 medium inoculated withS. sciurionE. balteatusin a greenhouse. (a) Average number of eggs on plants (N=100/zone) sprayed or not with the 863 medium (n=3). (b) Average number of eggs on plants (N=100/zone) sprayed or not with the 863 medium inoculated withS. sciuri(n=3). ***indicates significant difference atP<0.001 (one-way Anova). Error bars indicate standard errors. Figure 4: Effect of the 863 medium inoculated with S. sciuri on E. balteatus in a greenhouse. ( a ) Average number of eggs on plants ( N =100/zone) sprayed or not with the 863 medium ( n =3). ( b ) Average number of eggs on plants ( N =100/zone) sprayed or not with the 863 medium inoculated with S. sciuri ( n =3). ***indicates significant difference at P <0.001 (one-way Anova). Error bars indicate standard errors. 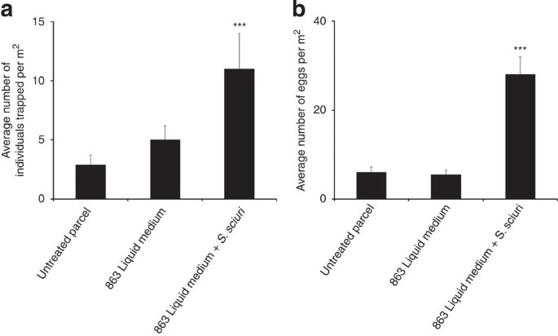Figure 5: Effect of the 863 medium inoculated withS. sciurionE. balteatusin a potato field. (a) Average number of individuals per m2trapped in the parcels sprayed or not with the 863 medium or with the 863 medium inoculated withS. sciuri(n=20). (b) Average number of eggs on plants in the parcels sprayed or not with the 863 medium or with the 863 medium inoculated withS. sciuri(n=20). ***indicates significant difference with the control atP<0.001 (one-way Anova). Error bars indicate standard errors. Full size image Figure 5: Effect of the 863 medium inoculated with S. sciuri on E. balteatus in a potato field. ( a ) Average number of individuals per m 2 trapped in the parcels sprayed or not with the 863 medium or with the 863 medium inoculated with S. sciuri ( n =20). ( b ) Average number of eggs on plants in the parcels sprayed or not with the 863 medium or with the 863 medium inoculated with S. sciuri ( n =20). ***indicates significant difference with the control at P <0.001 (one-way Anova). Error bars indicate standard errors. Full size image Although the bacterium S. sciuri was isolated from gut flora of aphids [42] , [43] and has been found previously in laboratory cultures of A. pisum [44] , [45] , the behaviours induced on hoverflies by the bacterium and its associated semiochemicals were unexpected. In the majority of cases, mediation of natural enemy behaviour has been found to be driven by plant or host volatiles. Our findings represent the first case of a host-associated bacterium driving prey location and ovipositional preference for the natural enemy through the emission of volatile compounds. Degradation and/or modifications of the large amounts of sugars and amino acids found in aphid honeydew could explain the detection of the volatile compounds identified from the honeydew: for example, 3-methyl-butanal and 2-methyl-butanal as well as their corresponding alcohols (3-methyl-1-butanol and 2-methyl-1-butanol) and their respective acids (3-methylbutanoic acid and 2-methylbutanoic acid) are known to be produced by direct modifications of the amino acids derived starter units, especially by Staphylococcus sp. bacteria [27] . Furthermore, the volatile compounds diacetyl (2,3-butanedione), acetoin (3-hydroxy-2-butanone), 3-methyl-3-buten-1-ol and benzeneethanol are typical fermentation-associated substances [27] , [46] . The flora of the aphid gut is partially acquired during probing on the host leaf surfaces or during feeding in the vascular tissues [45] , [47] . In this sense, several microorganisms were isolated from bean leaves [48] which could indicate that these microorganisms can be acquired by aphids. Indeed, small bacteria are able to pass through the stylets' food canal before adhering to the luminal face of intestinal epithelia [44] , [45] , [47] and finally being partially excreted in the honeydew. Because both S. sciuri and A. calcoaceticus were isolated from the pea aphid body and from the honeydew, the aphid itself may be considered as the source of the honeydew bacteria rather than free-living bacteria colonizing this excretory product. Consequently, these two bacteria could be considered as host-associated bacteria being partially excreted by the aphids. Furthermore, because S. sciuri has been found under natural conditions such as water, soil and grass samples [49] and also found in two natural aphid species in this study, it could be assumed that aphids can be considered a 'habitat' for these accessory bacteria acquired during probing [43] . Previously, S. sciuri was only identified under favourable conditions encountered in the laboratory cultures [42] , [43] , [44] , [45] , but our results show that this bacterium is present among natural aphid populations collected in field crops. The presence of honeydew on plant leaves constitutes an excellent growth medium promoting the rapid development of several microorganisms such as S. sciuri that are fairly widespread in nature [49] . Bacterial growth on honeydew and honeydew degradation are responsible for the emission of specific volatiles that are only emitted if a highly concentrated sugary medium such as aphid honeydew may allow the bacterial development. The produced volatiles could therefore be perceived by some insects, particularly those that feed on aphids. This strongly leads to speculate that natural enemies can evolve the ability to associate the presence of volatiles produced by bacteria living on honeydew with the presence of aphids and food. Staphylococcus spp. is known to produce many odorant volatiles [27] , but the interactions between S. sciuri and natural enemies of aphids have not been previously investigated. Our findings represent not only the first isolation of bacteria and the associated semiochemicals from the aphid honeydew, but also the identification of their attractive and ovipositional roles in these tritrophic interactions. With a growing interest in the use of natural enemies for crop protection, our results will prompt new studies that may lead to the use of S. sciuri and its associated semiochemicals for biological control against aphids. Rearing plants and insects In a climate-controlled room (16 h light photoperiod; 60±5% RH; 20±2 °C), the Vicia faba L. plants were grown in a mixture of vermiculite and perlite (1/1) and were infested with the aphid A. pisum (Harris). In the same climatic conditions, E . balteatus larvae were obtained from a mass production; the hoverflies were reared with sugar, pollen and water; and the oviposition was induced by the introduction of infested host plants in the rearing cage during 3 h. The complete life cycle took place on the host plants that were daily re-infested with aphids. Syrphid pupae were provided by Katz Biotech AG. Identification of honeydew and aphid bacterial contents To investigate the honeydew microflora, 20 μl of A. pisum honeydew were collected; several V. faba plants abundantly infested with aphids were placed 10 cm above an aluminium foil; and using microcapillaries of 10 μl volume, the honeydew droplets naturally falling on the aluminium sheet were directly collected in sterile conditions. To determine the aphid bacterial content, the whole bodies of 20 A. pisum adults that were surface-sterilized by dipping into 70% ethanol for 3 min, were washed in a 9 g l −l NaCl solution and then crushed in the same solution. For honeydew and crushed aphids, thus-obtained samples were then diluted and plated on the 868 agar medium (containing (per litre of distilled water) 1.7% of agar and 10 g each of glucose, yeast extract and casein peptone). Colonies were visible after 24 h of incubation at 25 °C and the strains were then isolated on the same medium. For the bacterial identification, genomic DNA was extracted from cells grown at 25 °C during the 48 h and PCR amplification of the 16S ribosomal DNA sequences was performed. Genomic DNA was purified by using Wizard Genomic DNA purification Kit (Promega). The primers used for PCR amplification of 16S ribosomal DNA sequences were the universal primers 16SP0 (5′-GAAGAGTTTGATCCTGGCTCAG-3′) and 16SP6 (5′-CTACGGCTACCTTGTTACGA-3′). The PCR mixture contained PCR Buffer, 2 mM MgCl 2 , 1 U of Taq polymerase (Fermentas) and each dNTP at a concentration of 20 mM (Promega). Running parameters were 25 cycles of 95 °C for 30 s, 55 °C for 30 s and 72 °C for 2 min; denaturing step was 5 min and the extension time at the end was 10 min. The PCR product was purified using GFX PCR DNA and Gel Band Kit (GE Healthcare) then sequenced using Big Dye v3.1 Kit and 3730 DNA analyser (Applied Biosystem). The sequences obtained (400–600 bp) were assembled with the program BIOEDIT. To ensure that the identified bacteria were not contaminants from the laboratory cultures, ten natural strains of aphids were collected in field crops and under greenhouse systems. Honeydew was collected from each aphid strain and the bacterial content was identified as described above. Identification of the honeydew volatile compounds The volatile collection was performed by SPME on the following different samples: an empty vial (control); 20 μl of crude honeydew; 20 μl of crude honeydew sterilized by filtration on a 0.2 μm filter using a 0.5 ml syringe; 20 μl of filtered crude honeydew, which was then inoculated with strains isolated from honeydew; 20 μl of the 863 medium (containing (per litre of distilled water) 10 g of each of the following substrates: glucose, yeast extract and casein peptone); 20 μl of the 863 medium inoculated with the two bacteria isolated from honeydew. After 24 h of bacterial growing, the reinoculated honeydews as well as the inoculated 863 media were controlled according to the optical density (OD) at 600 nm. The obtained OD were compared with the one measured with crude honeydew (OD=1.6). Five replications were performed per aliquots. The SPME volatile collection was conducted using an 85 μm carboxen-polydimethylosiloxane (Carboxen-PDMS, stableflex) (Supelco) coating fibre. Before each use, the fibre was conditioned at 300 °C for 1 h in a split-splitless GC injector. Volatile collections were performed at 20±1 °C during the 24 h. After each volatile collection, the SPME fibre was withdrawn from the vial and analysed by GC–MS. GC–MS analyses were carried out on an Agilent 6890N Network GC System coupled with an Agilent 5973 Network mass selective detector and equipped with a HP-5 (Agilent) capillary column (30 m×0.25 mm i.d., 0.25 μm film thickness). The oven temperature programme was initiated at 40 °C, held for 7 min and then raised first at 4 °C per min to 250 °C; then, it was held for 5 min and raised in the second ramp at 7 °C per min to 280 °C, and held for 1 min. Other operating conditions were as follows: carrier gas, He; with a constant flow rate of 1 ml per min; injector temperature, 260 °C; splitless mode. Mass spectra were taken at 70 eV. Mass range was from m/z 35 to 350 amu. The honeydew volatile components were identified by comparing their mass spectra fragmentation patterns with those stored in the Wiley275.L computer library. Furthermore, to validate the identification based on the mass spectral data, the GC retention times of the identified natural components were compared with the retention times of synthetic standards (more than 97% pure; Sigma-Aldrich). The relative proportion (%) of each identified chemical cue was calculated as followed: the area under the peak of the considered chemical cue was divided by the total peak area (corresponding to the sum of the areas of all sample-related peaks). Quantification of the semiochemicals of interest 3-methyl-2-butenal, butanoic acid and 2-methylbutanoic acid were carried out by comparing GC detector response (peak area) with a calibration curve developed using solutions containing known amounts of these chemicals (more than 97% pure; Sigma-Aldrich) ranging from 1 ng to 1 μg in iso-octane (Acros Organic), and analysed under analytical conditions identical to those of SPME analyses (five replications were performed). This method was used and described by Ming and Lewis [50] . Wind tunnel assays First, 150 μl of crude, filtered or reinoculated honeydew, or 150 μl of the 863 medium inoculated with S. sciuri (3×10 6 CFU per ml), or 150 μl of the 863 medium were sprayed (using a small glass sprayer) on plants (10-day-old V. faba plants, 10 cm high, 2 leaves). Second, the 15 identified volatile compounds (more than 97% pure; Sigma-Aldrich) were formulated in paraffin oil solution (10 μg μl −1 ). Rubber septa, placed near the stem of the plants, were filled with 100 μl of the solutions. Clean plants constituted the negative controls and the positive control consisted in plants infested with 10 A. pisum aphids. Ten E. balteatus (5 males and 5 females; 15–20 days old) were introduced into the tunnel 2 m downwind from the odour source. The wind tunnel was constructed of Plexiglas (L×W×H=2.4×0.8×0.6 m) and the experimental conditions were as follows: velocity of 0.4 m per second (laminar flow); T=20±2 °C; RH=60–70%; illumination=2,300 lux. The positions of individuals were observed every 20 min for 2 h, determining the percentage of individuals around the plants (less than 30 cm) (attraction), the percentage of individuals on the plant and the percentage of individuals remaining around the plants (less than 30 cm) during the 2 h (retention). The numbers of eggs laid on plants were noted after the 2 h of the experimentations. Two replications were performed for each tested lure. Percentage of individuals and number of eggs laid were analysed by generalized linear mixed models, the first one with a binomial error distribution, and the second with a Poisson error distribution. Statistical analyses were performed with R statistical software v2.10.1. Assays under greenhouse A compartment of the greenhouse (6×4×2 m) was divided into two zones in each of which 100 bean plants ( V. faba , 20 cm high; 4–5 leaves) were planted. In one of the two zones, plants were sprayed with the 863 liquid medium, or with the 863 medium inoculated with S. sciuri (3×10 6 CFU per ml) (150 μl per plant), whereas plants of the second zone were not treated. 50 gravid female hoverflies were dropped in the greenhouse and the numbers of eggs on the plants from each zone were noted after the 24 h. Treatments were switched to the opposite sides of the greenhouse to avoid differences in light, air flow, temperature and relative humidity, between the two parts of the greenhouse. Average temperature and relative humidity were, respectively, 24±2 °C and 60–70%. Three replications were performed. Average numbers of eggs per plant were compared by a one-way analysis of variance (Anova) (R statistical software v2.10.1.). Assays in the field In a potato field ( Solanum tuberosum var. Ditta) (50°30.565′N, 4°51.305′E), 20 parcels (1 m 2 ) randomly distributed in a 6 ha field were sprayed with 50 ml of the 863 medium or with 50 ml of the 863 medium inoculated with S. sciuri (3×10 6 CFU per ml) whereas 20 other parcels were untreated. In each parcel, a sticky trap (BugScan, Biobest) was placed to trap all the flying insects. Plants were not infested by aphids (visual observations). Parcels were separated by 30 m of untreated potato plants. Two days after the treatments, traps were removed and the numbers of trapped E. balteatus were noted. Syrphid eggs were counted in each parcel. Average numbers of individuals trapped per m 2 and average numbers of eggs per m 2 were compared by a one-way Anova (R statistical software v2.10.1. ). How to cite this article: Leroy, P. D. et al . Microorganisms from aphid honeydew attract and enhance the efficacy of natural enemies. Nat. Commun. 2:348 doi: 10.1038/ncomms1347 (2011).